Molecular mechanism of strigolactone perception by DWARF14 Strigolactones (SLs) are phytohormones that inhibit shoot branching and function in the rhizospheric communication with symbiotic fungi and parasitic weeds. An α/β-hydrolase protein, DWARF14 (D14), has been recognized to be an essential component of plant SL signalling, although its precise function remains unknown. Here we present the SL-dependent interaction of D14 with a gibberellin signalling repressor SLR1 and a possible mechanism of phytohormone perception in D14-mediated SL signalling. D14 functions as a cleavage enzyme of SLs, and the cleavage reaction induces the interaction with SLR1. The crystal structure of D14 shows that 5-hydroxy-3-methylbutenolide (D-OH), which is a reaction product of SLs, is trapped in the catalytic cavity of D14 to form an altered surface. The D14 residues recognizing D-OH are critical for the SL-dependent D14−SLR1 interaction. These results provide new insight into crosstalk between gibberellin and SL signalling pathways. The terpenoid, small-compound strigolactones (SLs) are plant hormones that regulate plant shoot branching [1] , [2] , which is an important agronomic trait that determines crop yields. In addition, SLs stimulate the germination of root parasitic weeds [3] , [4] that cause devastating crop damage [5] and induce hyphal branching in symbiotic arbuscular mycorrhizal fungi that promote the growth of host plants by capturing essential inorganic nutrients from the soil [6] , [7] , [8] . Owing to the importance of SLs in agriculture, the mechanism and signal transduction pathway of SLs have been extensively researched to provide a perspective on the broader SL functions. However, the mechanisms responsible for SL recognition by plants are poorly understood. SLs contain a structural core that consists of a tricyclic-lactone (ABC-ring) and a butenolide group (D-ring) that are connected via an enol ether linkage (compounds 1 − 4 ; Supplementary Fig. S1a ). In plants, SLs are synthesized from carotenoids through carlactone ( 4 ) (ref. 9 ), a butenolide-containing compound with SL-like biological activity, by a sequential reaction of several enzymes, including an iron-binding protein D27 (ref. 9 ), the carotenoid cleavage dioxygenases 7 and 8, and a cytochrome P450 protein MAX1 (refs 10 , 11 , 12 ) ( Supplementary Fig. S1b ). In addition, studies on a set of branching mutants of some plant species have indicated that the d14 and d3 / max2 / rms4 genes are closely related to a pathway downstream of SLs [1] , [2] , [13] , [14] ( Supplementary Fig. S1b ). D14 genes encode α/β-hydrolase family proteins [13] , [14] , [15] , [16] and their mutants exhibit a highly branched phenotype and are insensitive to SLs [13] , [14] . The d3/max2/rms4 mutants are also SL insensitive [1] , [2] . D3/MAX2/RMS4 genes encode members of the F-box-family protein [17] , [18] , [19] , [20] that participate in an Skp-cullin-F box (SCF) complex [18] and have diverse roles in the plant lifecycle [14] , [21] , [22] , [23] , [24] , [25] , [26] , [27] , [28] , [29] , [30] . Recently, it has been reported that petunia DAD2, an orthologue of rice DWARF14 (D14) protein, can hydrolyse the enol ether linkage of GR24 and interacts with PhMAX2A, a petunia orthologue of Arabidopsis MAX2 protein, indicating that the formation of the DAD2–PhMAX2A complex initiates an SCF-mediated signal transduction pathway [31] . However, it still remains unclear how the hydrolyzation of SLs induces the formation of the DAD2–PhMAX2 complex and what is/are the target(s) of the SCF complex. The Arabidopsis gibberellin (GA) biosynthetic mutant ga1-3 exhibits enhanced shoot branching, and the overexpression of GA 2-oxidase genes in rice, in which GA levels are reduced, promotes tillering [32] . These results suggest that GAs regulate branching together with or without SLs. The DELLA-family proteins are key negative regulators of GA signalling through interaction with growth promoting transcription factors, such as PIFs. DELLA proteins have recently been reported to upregulate jasmonate (JA) signalling by physically interacting with JAZs, repressors of JA signalling [33] . Further, JAZs reportedly inhibit DELLAs−PIFs interactions. Thus, JA inhibits plant growth by inducing the degradation of JAZs and restoring the interaction of DELLAs with PIFs [34] ( Supplementary Fig. S1c ). In addition, recent reports suggest that a transcription factor, which broadly regulates brassinosteroid signalling, BZR1, mediates growth response to GA via direct interaction with DELLAs [35] , [36] . These reports indicate that DELLAs have a role in regulating multiple signals. To investigate whether DELLAs mediate crosstalk between GA and SL signalling pathways, we explored the interaction between the rice D14 and the DELLA protein SLR1. Here we show that the rice D14 interacts with SLR1 in an SL-dependent manner, thus contributing to the negative regulation of GA signalling [37] ( Supplementary Fig. S1d ). Moreover, a series of crystallographic and biochemical studies suggest an advanced molecular mechanism of D14 in SL perception and signal transduction. Our results provide new insight into the crosstalk between the GA and SL signalling pathways. D14 interacts with the DELLA protein SLR1 To investigate whether D14 interacts with DELLA proteins, we performed a yeast two-hybrid (Y2H) assay using D14 as the bait and SLR1, the only DELLA protein in rice, as the prey in the presence of various SLs, including (±)-2′- epi -5-deoxystrigol (a racemic mixture of natural SLs (+)-2′- epi -5-deoxystrigol ( 1 ) and (−)-ent-2′- epi -5-deoxystrigol), (±)-GR24 (a racemic mixture of (+)-GR24 ( 2 ) and (−)- ent -GR24 ( 5 )), and (±)-2′- epi -GR24 (a racemic mixture of (+)-2′- epi -GR24 and (−)- ent -2′- epi -GR24). The result indicated that these SLs induced a D14–SLR1 interaction ( Fig. 1a ). When (−)- ent -GR7 ( 6 ) was added to the medium, this D14–SLR1 interaction was not observed, whereas when (−)- ent -2′- epi -GR7 ( 3 ), an enantiomer of (−)- ent -GR7 ( 6 ), was added to the medium, this interaction was clearly observed ( Fig. 1b ). Among the other tested SLs, 5,6-dihydro-(−)- ent -2′- epi -GR7 (dihydro-GR7, 7 ; Supplementary Fig. S2b ) also induced the interaction between D14 and SLR1, but 5,6,3′,4′-tetrahydro-(−)- ent -2′- epi -GR7 (tetrahydro-GR7, 8 ; Supplementary Fig. S2b ) did not induce the interaction ( Supplementary Fig. S2a ). The inhibitory effect of (−)- ent -2′- epi -GR7 ( 3 ) on the tiller bud outgrowth of rice was stronger than that of (−)- ent -GR7 ( 6 ) ( Fig. 1c ), indicating that the D14–SLR1 complex is formed in the presence of active SL forms. Similar results were obtained in the Y2H assay using dihydro-GR7 ( 7 , active form) and tetrahydro-GR7 ( 8 , less active form) ( Supplementary Fig. S2 ). The direct interaction between D14 and SLs was determined using a non-equilibrium gel-permeation technique and [5,6- 3 H]-5,6-dihydro-(−)- ent -2′- epi -GR7 (T 2 -GR7, 9 ; Fig. 2a ), a radioactive SL. The results showed that D14 bound T 2 -GR7 ( 9 ) and that the binding was replaced in the presence of excess unlabelled (±)-GR24 ( Fig. 2a ). The half-time for the association between D14 and T 2 -GR7 ( 9 ) was <1 min ( Fig. 2b ), indicating that the binding reaction occurs rapidly. Such rapid receptor-ligand binding was also reported for the OsGID1–GA association [38] . 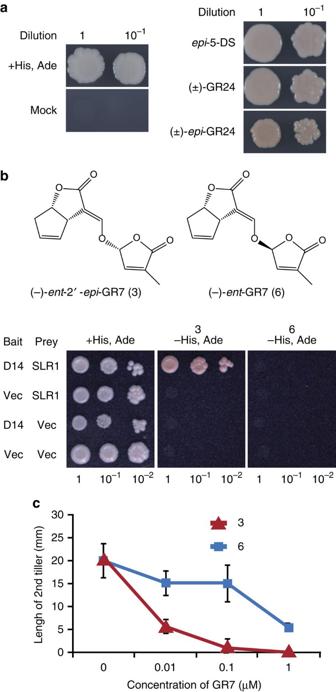Figure 1: Interaction between D14 and SLR1. (a) Growth of AH109 transformants with pGBK-D14 and pGAD-SLR1 on SD-His, Ade plates with various SLs.epi-5-DS: (±)-2′-epi-5-deoxystrigol. (±)-epi-GR24: (±)-2′-epi-GR24. (b) Structures of (−)-ent-2′-epi-GR7 (3) and (−)-ent-GR7 (6) and growth of AH109 transformants on an SD-His, Ade plate with or without 10 μM (−)-ent-2′-epi-GR7 (3) or (−)-ent-GR7 (6). (c) Length of second tillers of 3-week-old rice treated with (−)-ent-2′-epi-GR7 (3) or (−)-ent-GR7 (6) (mean±s.d.;n=5). Figure 1: Interaction between D14 and SLR1. ( a ) Growth of AH109 transformants with pGBK-D14 and pGAD-SLR1 on SD-His, Ade plates with various SLs. epi -5-DS: (±)-2′- epi -5-deoxystrigol. (±)- epi -GR24: (±)-2′- epi -GR24. ( b ) Structures of (−)- ent -2′- epi -GR7 ( 3 ) and (−)- ent -GR7 ( 6 ) and growth of AH109 transformants on an SD-His, Ade plate with or without 10 μM (−)- ent -2′- epi -GR7 ( 3 ) or (−)- ent -GR7 ( 6 ). ( c ) Length of second tillers of 3-week-old rice treated with (−)- ent -2′- epi -GR7 ( 3 ) or (−)- ent -GR7 ( 6 ) (mean±s.d. ; n =5). 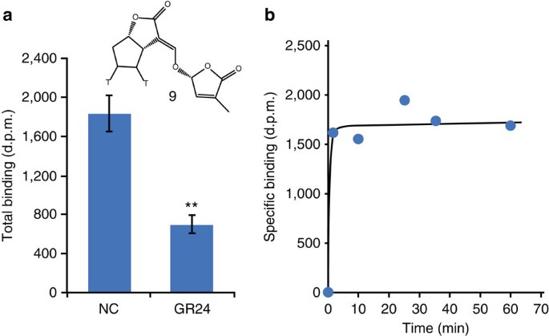Figure 2: SL-binding properties of D14 proteins. (a) Competition for T2-GR7 (9) binding to D14 by cold SLs (mean±s.d.,n=3). NC, no competitor. d.p.m., disintegrations per minute. **P<0.01 (Student’st-test) versus no competitor control. The structure of T2-GR7 (9) is shown as an inset. (b) Association rates of T2-GR7 (9) and D14. The specific binding of T2-GR7 (9) reached one-half of the maximum within 1 min (mean;n=2−3). Full size image Figure 2: SL-binding properties of D14 proteins. ( a ) Competition for T 2 -GR7 ( 9 ) binding to D14 by cold SLs (mean±s.d., n =3). NC, no competitor. d.p.m., disintegrations per minute. ** P <0.01 (Student’s t -test) versus no competitor control. The structure of T 2 -GR7 ( 9 ) is shown as an inset. ( b ) Association rates of T 2 -GR7 ( 9 ) and D14. The specific binding of T 2 -GR7 ( 9 ) reached one-half of the maximum within 1 min (mean; n =2−3). Full size image Subsequently, we performed a bimolecular fluorescence complementation (BiFC) analysis using chimeric proteins fused with split yellow fluorescent proteins (YFPs) to confirm whether the D14–SLR1 complex forms in vivo . Constructs for the expression of the fusion proteins, GFP–D14, nYFP–SLR1 and cYFP–D14, were transiently expressed in Arabidopsis protoplasts. The GFP–D14 fusion protein localized to the cytosol and the nucleus. A strong reconstituted YFP signal was observed demonstrating the nuclear interaction between D14 and SLR1 ( Fig. 3a ). This result is also consistent with the previous observations that DELLA proteins are localized to the nucleus [39] . 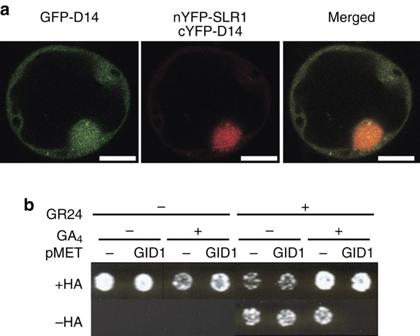Figure 3: D14–SLR1 interactionin plantaand the competition between the D14–SLR1 interaction and the GID1–SLR1 interaction. (a) BiFC analysis of the D14–SLR1 interaction. D14–GFP, cYFP–D14 and nYFP–SLR1 were expressed transiently in the protoplasts of Arabidopsis suspension-cultured cells. Scale bars, 10 μm. (b) Growth of AH109 transformants with pBridge-BDD14-MGID1 (or pBridge-BDD14) and pGAD-SLR1 on SD-His, Ade, Met plates with or without 10 μM (±)-GR24 and 1 μM GA4.When only (±)-GR24 was added to the growth medium, yeast colonies could grow independently of GID1 expression. In contrast, when both (±)-GR24 and GA3were added, the GID1-expressing yeast could not grow on the SD-His, Ade and Met medium. Figure 3: D14–SLR1 interaction in planta and the competition between the D14–SLR1 interaction and the GID1–SLR1 interaction. ( a ) BiFC analysis of the D14–SLR1 interaction. D14–GFP, cYFP–D14 and nYFP–SLR1 were expressed transiently in the protoplasts of Arabidopsis suspension-cultured cells. Scale bars, 10 μm. ( b ) Growth of AH109 transformants with pBridge-BDD14-MGID1 (or pBridge-BDD14) and pGAD-SLR1 on SD-His, Ade, Met plates with or without 10 μM (±)-GR24 and 1 μM GA 4 .When only (±)-GR24 was added to the growth medium, yeast colonies could grow independently of GID1 expression. In contrast, when both (±)-GR24 and GA 3 were added, the GID1-expressing yeast could not grow on the SD-His, Ade and Met medium. Full size image SLR1 has key roles as a negative regulator of GA signalling [37] and interacts with OsGID1 in GA-dependent manner ( Supplementary Fig. S1d ). To confirm whether the SL-dependent D14–SLR1 interaction is competitive with the GA-dependent OsGID1–SLR1 interaction, we established a yeast three-hybrid (Y3H) system; D14 was used as the bait, SLR1 was used as the prey and OsGID1 was used as a D14 competitor ( Fig. 3b ). When both (±)-GR24 and GA 4 were added, OsGID1-expressing yeast cells could not grow on the medium lacking L -histidine and adenine. This result indicates that the formation of the GR24-dependent D14–SLR1 complex is inhibited by the GA 4 -bound OsGID1, and the D14-interacting domain overlaps with the OsGID1-interacting domain in SLR1. D14−SLR1 interaction requires enzymatic activity of D14 The enzymes belonging to the α/β-hydrolase superfamily contain a nucleophile-histidine-acid catalytic triad, which is required to catalyse the hydrolytic cleavage of the substrates. The corresponding catalytic residues are conserved in D14 as Ser147 (nucleophile)-His297-Asp268 ( Supplementary Fig. S3 ). To evaluate the D14 catalysis of the hydrolytic cleavage of SLs, we observed the degradation of (±)-GR24 by D14 using an HPLC technique with a Chiralpak IA-3 column ( Fig. 4a ). Two peaks of (−)- ent -GR24 ( 5 ) and (+)-GR24 ( 2 ) (peaks A and B, respectively, in Fig. 4a ) were stably detected when (±)-GR24 was incubated for 1 h without D14. In contrast, the peak of (+)-GR24 ( 2 ) disappeared when (±)-GR24 was incubated with D14 for 1 h, whereas the peak of (−)- ent -GR24 ( 5 ) was stable. The peak of (−)- ent -GR24 ( 5 ) disappeared after overnight incubation with D14, indicating that (−)- ent -GR24 ( 5 ) could be a substrate for the hydrolytic cleavage by D14, whereas (+)-GR24 ( 2 ) is a more favourable substrate than (−)- ent -GR24 ( 5 ). These results indicate that D14 has the catalytic ability to hydrolyse SLs, which is consistent with the observations of DAD2 (ref. 31 ), and, to some extent, this catalysis is stereoselective. 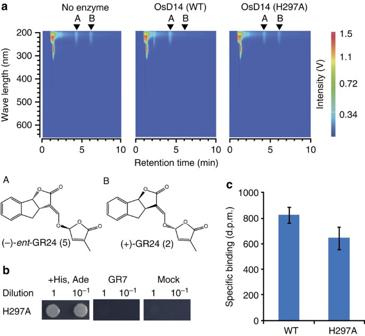Figure 4: Catalytic activity of D14 in the interaction with SLR1. (a) Enzymatic degradation of (±)-GR24 by D14. (±)-GR24 (10 μM) was incubated with or without purified D14 for 1 h at 37 °C. The reaction solutions were extracted with ethyl acetate, and the organic layer was subjected to HPLC analyses using a Chiralpak IA-3 column. Peaks A and B were confirmed to represent (−)-ent-GR24 (5) and (+)-GR24 (2), respectively, as described in the Methods section. The experiments were repeated three times with similar results. (b) Growth of AH109 transformants with pGAD-SLR1 and the wild-type or mutated D14 cDNA on pGBK-T7 on an SD-His, Ade plate with or without 10 μM (−)-ent-2′-epi-GR7 (3). (c) Comparison of the specific binding of T2-GR7 (9) to wild-type D14 and to H297A mutant D14 (mean±s.d.,n=3). Figure 4: Catalytic activity of D14 in the interaction with SLR1. ( a ) Enzymatic degradation of (±)-GR24 by D14. (±)-GR24 (10 μM) was incubated with or without purified D14 for 1 h at 37 °C. The reaction solutions were extracted with ethyl acetate, and the organic layer was subjected to HPLC analyses using a Chiralpak IA-3 column. Peaks A and B were confirmed to represent (−)- ent -GR24 ( 5 ) and (+)-GR24 ( 2 ), respectively, as described in the Methods section. The experiments were repeated three times with similar results. ( b ) Growth of AH109 transformants with pGAD-SLR1 and the wild-type or mutated D14 cDNA on pGBK-T7 on an SD-His, Ade plate with or without 10 μM (−)- ent -2′- epi -GR7 ( 3 ). ( c ) Comparison of the specific binding of T2-GR7 ( 9 ) to wild-type D14 and to H297A mutant D14 (mean±s.d., n =3). Full size image No interaction of DAD2 with PhMAX2A was observed by the mutation of the catalytic triad residues [31] . To evaluate the significance of the enzymatic reaction in the interaction between D14 and SLR1, we performed a mutational analysis of D14 using a Y2H system. A mutation in the catalytic residue His297 (H297A) decreased the enzymatic activity of D14 towards GR24 ( Fig. 4a ) and abolished the SLR1 interaction in both the presence and absence of (−)- ent -2′- epi -GR7 ( 3 ) ( Fig. 4b ). In addition, the competitive binding assay using T 2 -GR7 ( 9 ) showed that the H297A mutant was capable to bind (±)-GR24 ( Fig. 4c ). This result indicates that the catalytically inactive mutant could form a constitutive enzyme–substrate complex, which supports that the complex is not capable to interact with SLR1. Thus, the SL-dependent SLR1 interaction requires the enzymatic activity of D14 towards SLs. Moreover, we examined whether the enzymatic cleavages of substrates are required for the interaction between D14 and SLR1. We prepared several SL analogues (compounds 10 – 13 ; Supplementary Fig. S4a ), in which various moieties were linked to the D-ring by ether or ester bonds. 3,5-dimethoxybenzoyloxy D-ring ( 12 ) and anthracene-9-carbonyloxy D-ring ( 13 ) induced D14−SLR1 interaction at a concentration of 10 μM in the Y2H assay, although methoxy D-ring and acetoxy D-ring did not induce D14−SLR1 at this concentration. However, acetoxy D-ring ( 11 ) induced D14−SLR1 interaction at a high concentration (100 μM), whereas methoxy D-ring ( 10 ) did not ( Supplementary Fig. S4b ). These data correspond to the results of the bioassay on the tiller bud outgrowth ( Supplementary Fig. S4c ). The fact that all active chemicals possessed an ester bond and that methoxy D-ring was inactive in the Y2H and the tillering inhibition assay suggests that the enzymatic cleavage of substrates by D14 is important for the interaction between D14 and SLR1, and the ester link is susceptible to hydrolysis by D14. Consistent with this hypothesis, we observed the D14 catalysis of the hydrolytic cleavage of anthracene-9-carbonyloxy D-ring using an HPLC technique ( Supplementary Fig. S4d ). D14 forms a complex with D-OH to mediate SLR1 interaction On examination of the recent model of D14 activation, it is predicted that the formation of a reaction intermediate may induce structural changes that facilitate the interaction between D14 and its target proteins [31] , [40] . The crystal structure of D14 with a GR24-degradation intermediate, 2,4,4-trihydroxy-3-methyl-3-butenal, could propose the reaction mechanism for producing a hydroxy ABC-ring (ABC-OH) and a hydroxy D-ring (D-OH) from GR24 (ref. 41 ), although it remains unclear whether the intermediate complex functions as an active form of SL signalling and no significant structural changes are found between the overall structures of apo and the intermediate. When we tried to co-crystallize D14 with several SLs including (±)-GR24 and (−)- ent -2′- epi -GR7 ( 3 ) and to soak the substrates into D14 crystals, we solved the crystal structure of D14 complexed with a reaction product D-OH at a 2.10-Å resolution ( Fig. 5a ). In this experiment, the cavity of D14 in the crystal could be exposed to solvent ( Supplementary Fig. S5a,b ) and, therefore, a substrate and a reactive water molecule could access to the cavity even in the crystal. D-OH may be produced via the reported intermediate, 2,4,4-trihydroxy-3-methyl-3-butenal [41] from the soaked (−)- ent -2′- epi -GR7 ( 3 ) by an in-crystal activity of D14. This product is located at a site far from the catalytic triad residues and is surrounded by Val194, Ser270 and several aromatic residues, such as Phe186, Trp205, Tyr209 and Phe245 ( Fig. 5b ). These residues make favourable hydrophobic and/or van der Waals interactions with D-OH. In addition, the indole amine of Trp205 forms a hydrogen bond with the oxygen atom of the C2′ hydroxy group, which could arise from the catalytic reaction of D14, instead of a water molecule in the structure of apo D14 ( Supplementary Fig. S5 ). In the complex structure, D-OH functions as a plug for the catalytic cavity of D14 and induces a hydrophilic patch in an overall hydrophobic surface between the two α-helices (αA and αB) in the cap structure of D14 ( Fig. 5c ). 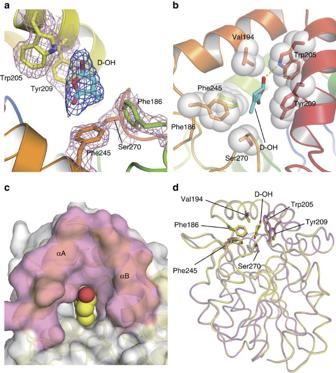Figure 5: D-OH recognition by D14. (a) Side view of D-OH bound to D14. D-OH and the surrounding residues are shown as a stick model along with the 2Fo−Fcelectron density coloured in blue and purple, respectively. (b) Binding site of D-OH. The residues surrounding D-OH are represented by a stick-and-sphere model. The dashed line shows a hydrogen bond between D-OH and the indole amine of Trp205. (c) Plug-like binding of D-OH to the catalytic cavity of D14. D-OH is shown using a sphere representation. (d) Superposed structure of apo and D-OH-bound D14. The crystal structures of apo and D-OH-bound D14 are shown as pink and yellow ribbon diagrams, respectively. D-OH and its surrounding residues are represented by stick diagrams. Phe245 is the only residue that moves (1.3 Å) towards D-OH. Figure 5: D-OH recognition by D14. ( a ) Side view of D-OH bound to D14. D-OH and the surrounding residues are shown as a stick model along with the 2 F o − F c electron density coloured in blue and purple, respectively. ( b ) Binding site of D-OH. The residues surrounding D-OH are represented by a stick-and-sphere model. The dashed line shows a hydrogen bond between D-OH and the indole amine of Trp205. ( c ) Plug-like binding of D-OH to the catalytic cavity of D14. D-OH is shown using a sphere representation. ( d ) Superposed structure of apo and D-OH-bound D14. The crystal structures of apo and D-OH-bound D14 are shown as pink and yellow ribbon diagrams, respectively. D-OH and its surrounding residues are represented by stick diagrams. Phe245 is the only residue that moves (1.3 Å) towards D-OH. Full size image Large structural differences were not observed between the apo and D-OH-bound D14 molecules, although the side chain of Phe245 was moved 1.3 Å towards D-OH ( Fig. 5d ). In addition, the Cα atoms of the αA- and αD-helices and the large loop connecting to the αA-helix were changed with the root mean square distance of >0.4 Å upon D-OH binding ( Supplementary Fig. S6 ). The Phe245 residue located on the αD-helix makes contact with the αA-helix and the loop. Therefore, these regions seem to be directly affected by the side-chain rearrangement of Phe245. In the previous study, it has been shown that the D14 orthologue DAD2 is destabilized in the reaction process of GR24 (ref. 31 ). The trypsin digestion assay showed that the D14 protein (wild type) was efficiently degraded when (±)-GR24 or (−)- ent -2′- epi -GR7 ( 3 ) was added in the reaction solution ( Supplementary Fig. S7 ). On the other hand, the degradation of the catalytically inactive H297A mutant was not affected by adding (±)-GR24 or (−)- ent -2′- epi -GR7 ( 3 ). These results are consistent with structural changes induced by D-OH binding. To evaluate the significance of D-OH binding in the interaction with SLR1, we performed a mutational analysis of D14 using a Y2H system. The SLR1 interactions in a GR7-dependent manner were lost when Phe186, Trp205 or Phe245 were mutated to alanine ( Fig. 6a ). These residues contact D-OH and/or form the hydrophobic surface observed on the cap structure. In addition, the side chain of Phe245 is rearranged on D-OH binding to slightly modify the local structure of the contact region with the residue, especially the αA-helix. The enzymatic activity towards GR24 was also decreased by the mutation of Trp205 as well as by the mutation of the catalytic residue, His297 ( Supplementary Fig. S8 ). As the interaction between D14 and SLR1 requires an enzymatic activity, the functional contribution of D-OH towards the D14−SLR1 interaction is unclear in these mutations. Trp205 may be essential to the binding of the GR24 molecule as well as the D-OH molecule in the cavity. In contrast, the F245A mutant showed a slightly lower enzymatic activity towards GR24 compared with that of wild-type D14 ( Supplementary Fig. S8 ), raising the possibility that the D14−D-OH complex mediates the interaction with SLR1 in which the D-OH-induced surface and/or structural change is crucial. Consistent with the importance of D-OH in the D14−SLR1 interaction, the addition of a high concentration of D-OH induced the interaction between D14 and SLR1 in the Y2H assay ( Fig. 6b ) and significantly suppressed the outgrowth of the tiller bud of a rice d27-1 mutant without affecting the plant height ( Fig. 6c ), indicating that the inhibition of the tiller outgrowth was not due to the toxic effect of a high concentration of D-OH. On the contrary, the addition of a high concentration of D-OH did not inhibit the outgrowth of the tiller bud of the SL-insensitive d3-1 mutant rice ( Supplementary Fig. S9 ). In agreement with the previous study [42] , the addition of a low concentration of D-OH (~10 μM) did not inhibit outgrowth of the tiller bud of rice and did not induce D14−SLR1 interaction in the Y2H assay. These results support that a reaction product D-OH induces the interaction between D14 and SLR1 as a mature form of SL to transmit the SL signalling ( Fig. 7 ). 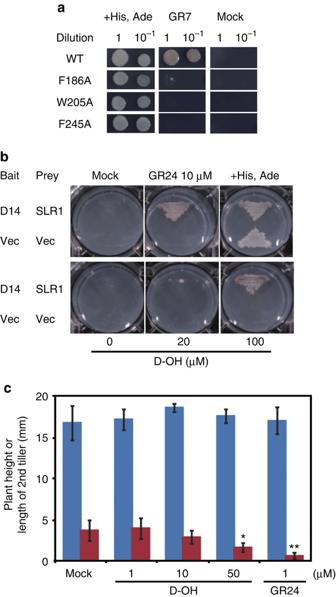Figure 6: Effects of D-OH in SLR1 interaction and in the outgrowth of tiller buds. (a) Growth of AH109 transformants with pGAD-SLR1 and the wild-type or mutated D14 cDNA on pGBK-T7 on an SD-His, Ade plate with or without 10 μM (−)-ent-2′-epi-GR7 (3). (b) Growth of AH109 transformants on an SD-His, Ade plate with or without D-OH. (c) Inhibition of the growth of second tiller buds by D-OH. The plant height (blue) and length of the second tillers (red) of 3-week-old rice plants that were treated with D-OH or (±)-GR24 (mean±s.d.;n=6) are shown. *P<0.05 and **P<0.01 (Student’st-test) versus non-treated control. Figure 6: Effects of D-OH in SLR1 interaction and in the outgrowth of tiller buds. ( a ) Growth of AH109 transformants with pGAD-SLR1 and the wild-type or mutated D14 cDNA on pGBK-T7 on an SD-His, Ade plate with or without 10 μM (−)- ent -2′- epi -GR7 ( 3 ). ( b ) Growth of AH109 transformants on an SD-His, Ade plate with or without D-OH. ( c ) Inhibition of the growth of second tiller buds by D-OH. The plant height (blue) and length of the second tillers (red) of 3-week-old rice plants that were treated with D-OH or (±)-GR24 (mean±s.d. ; n =6) are shown. * P <0.05 and ** P <0.01 (Student’s t -test) versus non-treated control. 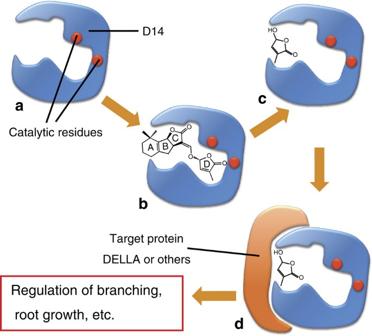Figure 7: A model of SL recognition and SL hydrolysation and the regulation of SL-induced signal transduction by D14. (a) The empty form of D14. (b) SL-bound D14. (c) SL is catabolized by D14, and D-OH is produced. D-OH then remains at the aperture area of the binding cavity of D14. (d) The hydrophobic surface of the cap structure of D14 is recognized by a target protein, such as SLR1, and the D14-SL-target protein complex modulates downstream signalling. (+)-5-deoxystrigol was shown in this model as a representative of natural SLs. Full size image Figure 7: A model of SL recognition and SL hydrolysation and the regulation of SL-induced signal transduction by D14. ( a ) The empty form of D14. ( b ) SL-bound D14. ( c ) SL is catabolized by D14, and D-OH is produced. D-OH then remains at the aperture area of the binding cavity of D14. ( d ) The hydrophobic surface of the cap structure of D14 is recognized by a target protein, such as SLR1, and the D14-SL-target protein complex modulates downstream signalling. (+)-5-deoxystrigol was shown in this model as a representative of natural SLs. Full size image Until now, D14 proteins were known to hydrolyse the enol ether linkage of SLs to produce ABC-OH and D-OH [41] and function in SL signalling [31] , but the mechanism for how SL perception is converted to SL signal transduction has not been clarified. Our results raise the possibility that D-OH induces the D14−SLR1 interaction and acts as an active branching inhibitor. In SLs and in compounds with SL-like biological activities, the D-ring unit and the enol ether section (>C=CH-O-) are common structures, whereas other moieties are rather flexible ( Supplementary Fig. 1a ). In addition, active SLs are catabolized by D14 and a reaction product D-OH is trapped in the cavity of D14. On the basis of these findings, we propose an advanced molecular mechanism of D14 in which D-OH functions as a mature form of SL to transmit the SL signalling ( Fig. 7 ): D14 functions in the conversion of SLs to the bioactive form D-OH and participates in SL signalling as a complex with D-OH by interacting with the target proteins such as SLR1. The addition of D-OH alone at the same concentration as the addition of other active SLs did not induce a D14–SLR1 interaction in the Y2H assay ( Fig. 6b ) and did not inhibit the tillering of the d27-1 mutant ( Fig. 6c ). Although further structural and biochemical experiments are needed, proper localization of D-OH in the aperture of the binding cavity of D14 may require the prior binding of SL followed by hydrolytic cleavage to produce D-OH. Alternatively, D-OH may not be transported and/or incorporated efficiently into the nuclei in plants. GA is received by the GA receptor GID1, which promotes the formation of the GA–GID1–DELLA protein complex. This complex is then recognized by the SCF SLY1/GID2 complex, which recruits DELLA proteins for proteasomal degradation [33] ( Supplementary Fig. 1c ). As GID1 and D14 are members of the α/β-hydrolase family and SLY1/GID2 and MAX2/D3 are members of the F-box family, D14 and MAX2/D3 are assumed to function in SL signalling in a manner similar to that of GID1 and SLY1/GID2 in GA signalling, and our results suggest that DELLA proteins are potential candidates for the target of the D14–MAX2/D3 complex ( Fig. 7 ). Direct interactions of DELLA proteins with other hormone signalling factors, such as JAZs and BZR1, have recently been reported to mediate the crosstalk between GA and JA signalling [33] , [34] , and between GA and brassinosteroid signalling [35] , [36] , respectively, indicating a pivotal role of DELLAs in regulating multiple signals. Our results suggest that the D14−DELLA interaction mediates the crosstalk between GA and SL signalling pathways. However, although both SL and GA repress the elongation of tillering buds, each hormone has distinct functions. For example, it is well known that the treatment of GA results in elongation of shoots, although the SL treatment does not cause the shoot elongation. Identification of factors involved in the D14–DELLA complex, such as PIFs in the JAZ–DELLA interaction, under various environmental and developmental situations will provide a better understanding of the mechanisms for the commonality and difference of actions of these hormones in response to environmental and plant developmental processes. Our model of the SL perception by D14 explains why a wide variety of natural SLs and analogues can exert their activity as branching inhibitors; the D-ring moiety of SLs is essential for hormonal activity [42] . Although SLs also function in arbuscular mycorrhizal fungi hyphal branching and in seed germination of parasitic plants, structure–activity relationships are different among individual organisms [4] , [8] , [42] , suggesting that each organism uses a distinct SL recognition system. The identification of SL perception mechanisms in different organisms would provide further information. Taken together, our findings contribute to the development of novel SL analogues and SL-signalling inhibitors for unveiling further details of SL signalling and for controlling plant growth and protecting crops from parasitic weeds to increase crop yields. Plant materials and growth conditions An SL-deficient d10-1 and d27-1 mutants of the Japonica-type rice cultivar ( Oryza sativa L. cv. Shiokari) was used in this study. Rice plants were grown as described previously [43] with some modifications. Germinated seeds were transferred into hydroponic culture medium [2] that was solidified with 0.6% agar and cultured at 25 °C under fluorescent white light with a 16-h light/8-h dark photoperiod for 6 days. Each seedling was transferred to a glass vial containing 12 ml of a sterilized hydroponic culture solution with or without chemicals and grown under the same conditions for 6 days. Plasmid construction All of the PCR primers used for plasmid construction are listed in Supplementary Table S1 . For the Y2H assay, pGADT7 (Clontech) and pGBK-T7 (Clontech) were used as the expression vectors. The D14 open reading frame fragment was amplified from total complementary DNA from rice seedlings by standard PCR with the D14-5- Eco RI and D14-3- Bam HI primers and cloned into the Eco RI- Bam HI site of the pGBK-T7 vector to construct pGBK-D14. Site-directed mutagenesis was performed by using the PrimeSTAR mutagenesis basal kit (Takara Bio Inc.) with pGBK-D14 as a template and the following primer sets: F186A-5 and F186-3 for pGBK-D14 F186A , W205A-5 and W205A-3 for pGBK-D14 W205A , F245A-5 and F245A-3 for pGBK-D14 F245A , and H297A-5 and H297A-3 for pGBK-D14 H297A . The SLR1 open reading frame fragment was amplified with the SLR1f and SLR1r primers and cloned into the Nde I- Eco RI site of the pGADT7 vector to construct pGAD-SLR1. To prepare the purified D14 proteins, the D14 cDNA fragment (residues 54−318) from rice was inserted into the pET-49b expression vector (Novagen). The fusion proteins contained a GST-tag at the amino terminus and an HRV3C protease site between GST and D14. To construct vectors for the BiFC assay, the N-terminal (1−154 a.a.) and carboxy-terminal (155−239 a.a.) fragments of enhanced YFP (eYFP; Clontech) were amplified by standard PCR using the following primer sets: eYFP-N0-f and eYFP-N0-r for eYFP 1-154 (N0 fragment) and eYFP-MC-f and eYFP-MC-r for eYFP 155–238 with methionine at its N terminus (MC fragment). The N0 and MC fragments were inserted into pUGW0 (ref. 44 ) at Aor 51HI sites to produce nYFP/pUGW0 and cYFP/pUGW0, respectively. To construct entry clones, the D14 and SLR1 fragments were amplified by two-step adaptor PCR as described by the manufacturer (Invitrogen). The templates were pGBK-D14 and pGAD-SLR1, and the following primer sets were used for the first PCR reaction: attB1-D14 and attB2-D14 for D14, and attB1-SLR1 and attB2-SLR1 for SLR1. The second PCR was performed with the attB1 and attB2 adaptor primers, and the amplified product was then inserted into pDONR221 via a BP reaction, as described by the manufacturer (Invitrogen) to construct pENTR-D14 and pENTR-SLR1. The DNA fragments from pENTR-D14 and pENTR-SLR1 were transferred into cYFP/pUGW0 and nYFP/pUGW0, respectively, via an LR reaction as described by the manufacturer (Invitrogen). Y2H and Y3H assays The Matchmaker Two-Hybrid System (Clontech) was used for the Y2H assay. pGBK-D14 served as the bait and pGAD-SLR1 served as the prey. Saccharomyces cerevisiae AH109 strains that were transformed with the bait and prey plasmids were grown in liquid media for 2 days, and the cell cultures were adjusted to OD 600 =10. Plate assays (synthetic defined (SD)-His, Ade) were performed according to the manufacturer’s protocol, with the modification that the plate media either did or did not contain SLs. For the Y3H assay, the yeast strains AH109 and Y187 and the plasmids pGADT7 and pBridge were obtained from Takara Bio Inc. pBridge-BDD14-MGID1 was constructed by fusing D14 cDNA with the GAL4-BD domain and inserting GID1 cDNA into the site downstream of pMET1. Strain Y187 was transformed with the pBridge vector harbouring BDD14 and pMET::GID1 or BDGID1 alone and selected on SD media lacking L -tryptophan (SD-Trp). Strain AH109, harbouring pGADT7–SLR1, grew on SD media lacking L -leucine and L -methionine (SD-Leu, Met). By mating both strains, the transformants carrying both plasmids (pBridge and pGADT7–SLR1) were selected on SD-Trp, Leu and Met. For the assay, the transformants were incubated on SD-Trp, Leu and Met media that lacked adenine hemisulphate and L -histidine but contained 3-aminotriazole. SL-binding assay For the SL-binding assay, [5,6- 3 H]-5,6-dihydro-(−)- ent -2′- epi -GR7 (T 2 -GR7, 9 ) was used as the radioactively labelled GR7. This labelled GR7 was synthesized with the help of Institute of Isotopes Co., Ltd (Budapest, Hungary). In vitro assays for SL binding were performed according to the method for the GA-binding assay [38] with some modifications. A total of 2 μg of the purified OsD14 protein was added to 300 μl of PBS buffer, and each sample was incubated with 100 μl of T 2 -GR7 ( 9 ; 1.13 nmol) in the presence of 442-fold excess of unlabelled (±)-GR24 (500 μM) for nonspecific binding or in the absence of excess unlabelled GR24 for total binding. Afterwards, 100 μl of the mixture was fractionated on a NAP-5 column (GE Healthcare). After discarding a void volume of PBS eluate (600 μl), a 200-μl fraction was collected, and its radioactivity was measured. The specific binding activity was calculated by subtracting the nonspecific binding from the total binding. BiFC assay For the BiFC assay, an Arabidopsis suspension culture was transiently transformed according to methods that were described previously [45] . The transformed cells were observed with a confocal laser microscopes. Multicolour observations were performed with an LSM710 confocal microscope (Carl Zeiss), as described previously [46] , [47] . A. thaliana -cultured cells were placed on eight-well multitest glass slides (MP Biomedicals) and covered with a 0.12–0.17-mm-thick coverslip (24 × 60 mm; Matsunami). The acquired images were analysed with the IMAGE J software program (National Institutes of Health). Protein preparation Rosetta (DE3) cells (Novagen) transformed with the expression vector for D14 were grown in Luria-Bertani broth at 37 °C to an OD 600 of ~0.6 and induced with 0.2 mM isopropylthio-β-galactoside at 25 °C for 16 h. The cells were collected and resuspended in extraction buffer (20 mM Tris–HCl (pH 8.5), 500 mM NaCl and 1 mM dithiothreitol (DTT)), which included 10% glycerol for D14. After sonication on ice, the lysate was centrifuged at 40,000 g in an Avanti J-E rotor (Beckman Coulter) for 30 min at 4 °C, and the supernatant was loaded onto a disposable polypropylene column packed with glutathione Sepharose 4B resin (GE Healthcare). The column was washed with the extraction buffer. On-column cleavage was performed overnight at 4 °C by adding HRV3C protease, and the target protein was eluted with each elution buffer as follows: 20 mM MES-NaOH (pH 6.5), 150 mM NaCl, 10% glycerol and 1 mM DTT. After the eluted product was diluted fourfold in elution buffer lacking NaCl, D14 was further purified using a Resource S column (GE Healthcare). D14 was eluted from a column with a 75−500-mM NaCl gradient in 20 mM MES-NaOH (pH 6.5), 10% glycerol and 1 mM DTT. Crystallization The purified protein was concentrated to 6.5 mg ml −1 in buffer containing 20 mM MES-NaOH (pH 6.5) and 0.5 M arginine hydrochloride. The D14 crystals were grown in sitting drops at 4 °C by vapour diffusion. The reservoir solution contained 0.1 M HEPES (pH 7.5), 8% PEG20000, and 2% 1,4-dioxane. Drops were prepared by mixing 0.8 μl of purified protein with 0.8 μl of reservoir solution. Crystals of ~100 μm in length appeared within 3 days. The crystals were soaked in the reservoir solution containing 0.2 M (−)- ent -2′- epi -GR7 ( 3 ) to obtain the protein–ligand complex. Data collection and structure determination The crystals were transferred into a reservoir solution containing 22% ethylene glycol before they were flash frozen in liquid nitrogen. X-ray diffraction data from a D14 crystal were collected on the AR-NE3A beamline at Photon Factory (Tsukuba, Japan). For a crystal of the protein–ligand complex, a diffraction data set was collected using an in-house X-ray diffractometer (Rigaku FR-E rotating-anode X-ray generator with R-AXIS VII imaging-plate detector). The diffraction images were integrated and scaled using the XDS package [48] . Molecular replacement was performed by using the CCP4 program Molrep with the Bacillus subtilis stress-response regulator RsbQ (PDB: 1WOM) [49] as the initial model. Coot [50] was used to manually fit the protein models. Model refinement was performed with the CCP4 program Refamc5 [51] . Most of the residues in the refined structures were in the most favourable region of the Ramachandran plot, and no residue was in the disallowed resign based on PROCHECK [52] (D14: residues in most favourable region, 97.1% and residues in allowed region, 2.9%; D14−D-OH complex: residues in most favourable region, 97.0% and residues in allowed region, 3.0%). The statistical analyses of the data sets and refined structures are listed in Table 1 . Table 1 Data collection and refinement statistics. Full size table Enzymatic in vitro assays The D14 in vitro assays were performed in a total volume of 1 ml of PBS buffer containing 10 μM (±)-GR24. Purified D14 was added at a final concentration of 12 μg ml −1 and incubated for 16 h at 37 °C. Next, 100 mg of NaCl was added to each reaction solution, and the reaction solutions were extracted with 400 μl of ethyl acetate three times. The organic layers were combined and dried in vacuo and dissolved in 15 μl of ethyl acetate. For each layer, 10 μl was applied to the HPLC analyses. The normal-phase chromatographic separation was performed on a Jasco HPLC system that was equipped with an HPLC pump of model PU 1580 (Jasco) and a photodiode array detector MD1505 (Jasco), and was controlled by the ChromNAV (Ver. 1.16.02) software program (Jasco). The analytical column was a Chiralpak IA-3 column (Φ 2.1 × 150 mm, Daicel) or a Chiralpak AD column (Φ 2.1 × 150 mm, Daicel). The analytes were eluted under isocratic conditions using 85% n -hexane and 15% ethanol at a flow rate of 0.5 ml min –1 . The chiral separation of (±)-GR24 was performed with a Chiralpak AD column, and each purified enantiomer was applied to the HPLC with a Chiralpak IA-3 column. We found that the compounds were eluted from a Chiralpak IA-3 column with the same order of elution as from a Chiralpak AD column. By comparing these data with the previously reported data using Chiralpak AD-H by Akiyama et al. [8] , it was confirmed that peak A represented (−)- ent -GR24 ( 5 ) and peak B represented (+)-GR24 ( 2 ). Trypsin digestion assay Purified D14 protein, which was dissolved in a solution containing 20 mM Tris–HCl (pH 8.0) and 0.1% dimethylsulphoxide at the final concentration of 5 μM, was incubated in the absence or presence of 10 μM (±)-GR24 or 10 μM (−)- ent -2′- epi -GR7 ( 3 ) at 4 °C for 15 min. The D14 solution was mixed with a trypsin solution containing 1 mg ml −1 trypsin, 1 mM HCl and 2 mM CaCl 2 by the volume ratio of 500:3 and was then incubated at 4 °C for 0, 1, 2, 4, 8, 12 or 24 h. The proteolysis reaction was stopped by mixing with 0.1 mM phenylmethanesulfonyl fluoride and SDS–PAGE sample buffer. The digested proteins were analysed by SDS–PAGE and Coomassie Brilliant Blue G-250 stain. Preparation of chemicals GR24 and GR7 were prepared as described previously [53] . SL analogues (compounds 10 − 13 ; Supplementary Fig. S4a ) were prepared according to the previously described reaction [54] . Among them, we synthesized two novel compounds as follows. 4-methyl-5-oxo-2,5-dihydrofuran-2-yl 3,5-dimethoxybenzoate (3,5-dimethoxybenzoyloxy D-ring) ( 12 ). In a 50-ml flask with a magnetic stir bar, potassium carbonate (0.18 g, 1.0 mmol) and tetra- n -butylammonium bromide (0.32 g, 1.0 mmol) were dissolved in a mixture of CH 2 Cl 2 (2 ml) and H 2 O (3 ml). Into this solution, 3,5-dimethoxybenzoic acid (0.35 g, 1.9 mmol) and 5-bromo-3-methyl-2(5H)-furanone (0.17 g, 1.0 mmol) in CH 2 Cl 2 (2 ml) were added and the mixture was stirred vigorously at room temperature for over 10 h. The reaction mixture was added to CH 2 Cl 2 and washed with brine, and the organic layer was dried over Na 2 SO 4 , and then filtered and concentrated in vacuo . The residue was purified by silica gel column chromatography and the resulting solid was recrystallized from ethanol/hexane to give 3,5-dimethoxybenzoyloxy D-ring ( 12 ) as a white solid. TLC (ethanol:hexane, 1:2 v/v): R f =0.47; 1 H NMR (500 MHz, CDCl 3 ): δ 7.17 (2H), 7.10(1H), 7.03(1H), 6.69(1H), 3.83(6H), 2.04(3H). 13 C NMR (125.65 MHz CDCl 3 ): δ 171.1 (C1), 164.6 (C1), 160.8 (2C), 142.1 (1C), 134.6 (1C), 130.2 (1C), 107.6 (2C), 106.8 (1C), 93.2 (1C), 55.6 (2C), 10.6 (1C). HRMS ( m / z ): [M+H] + calcd. for C 14 H 15 O 6 , 279.0863; found, 279.0874. 4-methyl-5-oxo-2,5-dihydrofuran-2-yl anthracene-9-carboxylate (anthracene-9-carbonyloxy D-ring) ( 13 ). In a 25-ml flask with a magnetic stir bar, sodium hydride (60%, dispersion in paraffin liquid, 0.05 g, 1.2 mmol), tetrahydrofuran (THF, 3 ml) and anthracene-9-carboxilic acid (0.44 g, 2.0 mmol) in THF (3 ml) were added and stirred. 5-bromo-3-methyl-2(5H)-furanone (0.17 g, 1.0 mmol) in THF (2 ml) was added and the mixture was stirred vigorously at room temperature for 4 h. The reaction mixture was added to CH 2 Cl 2 and washed with brine, and the organic layer was further extracted with brine twice. The combined aqueous layers were washed with ethanol twice and dried over Na 2 SO 4 , and then filtered and concentrated in vacuo . The residue was purified by silica gel column chromatography and the resulting solid was recrystallized from ethanol/hexane to give anthracene-9-carbonyloxy D-ring ( 13 ) as a yellow solid. TLC (ethanol:hexane, 1:2 v/v): R f =0.48; 1 H NMR (500 MHz, CDCl 3 ): δ 8.58 (1H), 8.09 (2H), 8.04 (2H), 7.59 (2H), 7.51 (2H), 7.46 (1H), 7.08 (1H), 2.01 (3H). 13 C NMR (125.65 MHz, CDCl 3 ): δ 171.0 (1C), 167.8 (1C), 141.8(1C), 134.9 (1C), 130.8 (2C), 130.5 (2C), 128.7 (3C), 127.6 (2C), 125.6 (2C), 125.1 (1C), 124.6 (2C), 93.0 (1C), 10.7 (1C). Accession codes. The structure coordinates and structural factors have been deposited in the Protein Data Bank under accession codes 3VXK (D14) and 3WIO (D14−D-OH complex). How to cite this article: Nakamura, H. et al. Molecular mechanism of strigolactone perception by DWARF14. Nat. Commun. 4:2613 doi: 10.1038/ncomms3613 (2013).